Plasmonic beaming and active control over fluorescent emission Nanometallic optical antennas are rapidly gaining popularity in applications that require exquisite control over light concentration and emission processes. The search is on for high-performance antennas that offer facile integration on chips. Here we demonstrate a new, easily fabricated optical antenna design that achieves an unprecedented level of control over fluorescent emission by combining concepts from plasmonics, radiative decay engineering and optical beaming. The antenna consists of a nanoscale plasmonic cavity filled with quantum dots coupled to a miniature grating structure that can be engineered to produce one or more highly collimated beams. Electromagnetic simulations and confocal microscopy were used to visualize the beaming process. The metals defining the plasmonic cavity can be utilized to electrically control the emission intensity and wavelength. These findings facilitate the realization of a new class of active optical antennas for use in new optical sources and a wide range of nanoscale optical spectroscopy applications. Optical antennas based on metal nanostructures have recently gained significant popularity for their unique ability to concentrate light into a deep-subwavelength volume [1] , [2] . They hold great promise for many emerging applications requiring tight confinement of optical fields, including sensors, photovoltaics, high-speed photodetectors and non-linear optics. Nanometallic antennas have also been used to tailor the excitation and emission processes of nearby fluorescent molecules or quantum dots (QDs) [3] , [4] , [5] , [6] . Strong local field concentration near illuminated metallic nanostructures is known to result in large excitation enhancements of quantum emitters [7] . Moreover, such particles can substantially enhance the local density of optical states and control the flow of light out of the emitter into free space. For example, metallic monopole and Yagi-Uda antennas have recently been used to redirect and shape the angular emission distribution of single molecules [8] , [9] . Currently, antenna structures that can produce one or more highly collimated optical beams from multiple quantum emitters and allow for electrical control over their emission properties are still lacking. The importance of the development of such antenna structures cannot be underestimated as fluorescence processes have a central role in many important applications, including optical spectroscopy techniques, biodetection, photochemistry and lighting. In parallel with the studies on radiative decay engineering with antennas, there is a growing body of work on shaping optical beams (for example, from a light-emitting diode or laser) with the use of patterned metal or dielectric films [10] , [11] , [12] , [13] . This line of research is aimed at realizing desirable beam properties without the use of bulky optical components. Here, we combine advances in the fields of radiative decay engineering and beam shaping to realize a new type of active optical antenna. The antenna enables unparalleled narrow angle collimation of fluorescent emission from a large number of quantum emitters placed in a nanoscale region; this goes beyond previous antenna designs that aim to produce collimated beams, which were limited in their use as they only efficiently couple to a single or a very limited number of emitters. The proposed structures also feature very relaxed fabrication tolerance levels compared with previous antenna designs and the placement of emitters is easy to accomplish. By simulating and optically imaging this flow of light, new intuition is gained about the operation of optical antennas as compared with traditional far-field measurements of the angular distribution of the emission intensity. Our work also builds and expands on previous studies based on the use of metal gratings (without a central slit) to direct emission from quantum emitters [14] , [15] , [16] . Finally, the proposed antenna architecture allows for electrical manipulation of QD emission. To illustrate this, we demonstrate active electrical control by exploiting the quantum-confined Stark effect and luminescence quenching. The unmatched, combined directional and electrical control over the emission of a large number of quantum emitters opens up a broad range of new opto-electronic and nanoscale spectroscopy applications for plasmonic antennas. 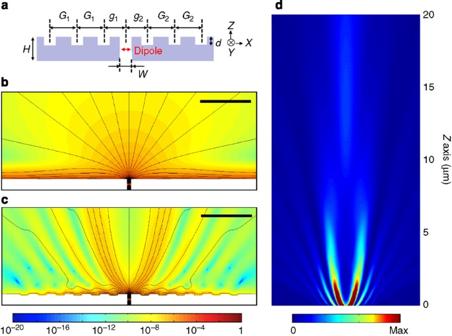Figure 1: Plasmonic beaming of the fluoresence from a quantum emitter. (a) Schematic of a plasmonic antenna consisting of a slit in a metal film (grey) that is surrounded by an engineered grating. An oriented, electrical dipole emitter is placed in the centre of the slit. The geometrical parameters that require careful optimization to enable beaming of the fluorescence are defined in the figure. (b) Simulation of the flow of light from an emitter in a slit onto a smooth metal surface in the form of surface plasmon polaritons. (c) Power flow image for the case where the central slit is flanked by an array of optimized grooves. (d) Plot showing the formation of a collimated far-field beam. The magnitude of the local power flow is shown in a logarithmic colour scale inbandc, but in linear colour scale ind. The black scale bar inbandcis 1 μm. The physics behind plasmonic beaming of fluorescent emission Figure 1a shows a schematic of the type of structure used in our experiments. It shows a nanoscale slit cut through a metal film surrounded by a carefully engineered miniature grating. We placed a large number of QDs (typically 10 2 –10 3 ) inside the slit and used the patterned metal structure to beam their emission. The physics involved in the optical beaming can most easily be understood by first considering a single, horizontally oriented dipole placed in the centre of the slit structure (as shown). From our previous studies, we determined that the emission from such a dipole very efficiently couples to a single, well-defined metal–dielectric–metal or 'gap' surface plasmon polariton (SPP) mode, which can be viewed as a special type of light wave [17] , [18] . Dipoles located in different, less symmetric positions inside the slit also preferentially couple to the same mode. The excited gap SPPs are known to very efficiently couple to planar SPPs that carry energy away from the slit along the metal surface [19] , [20] . It is thus expected that a good fraction of the dipole emission first couples to gap SPPs and then 'spills' onto the surface in the form of planar SPPs. Figure 1b confirms this expectation by showing the flow of light from the emitter onto the metal surface; shown are the streamlines associated with the time-averaged Poynting vector, as explained in the Supplementary information . A thoughtfully engineered array of grooves can now be used to efficiently decouple the planar SPPs to form a beam with a narrow angular divergence. The details of the complex decoupling process are shown in Figure 1c and the final beam formation in the far field is shown in Figure 1d . Figure 1: Plasmonic beaming of the fluoresence from a quantum emitter. ( a ) Schematic of a plasmonic antenna consisting of a slit in a metal film (grey) that is surrounded by an engineered grating. An oriented, electrical dipole emitter is placed in the centre of the slit. The geometrical parameters that require careful optimization to enable beaming of the fluorescence are defined in the figure. ( b ) Simulation of the flow of light from an emitter in a slit onto a smooth metal surface in the form of surface plasmon polaritons. ( c ) Power flow image for the case where the central slit is flanked by an array of optimized grooves. ( d ) Plot showing the formation of a collimated far-field beam. The magnitude of the local power flow is shown in a logarithmic colour scale in b and c , but in linear colour scale in d . The black scale bar in b and c is 1 μm. Full size image It is worth discussing the uniqueness of this scheme. In previous studies on beaming of external optical beams [10] , [11] , [12] , [13] , the goal was to obtain the highest possible throughput of incident source light through an aperture, while maintaining desired beaming properties. Here, the aperture serves as a nanoscale optical cavity that can be engineered to efficiently direct the emission of emitters placed inside the cavity. Furthermore, in contrast to previous directional antenna designs [9] , [21] , [22] , [23] , [24] , [25] , this structure now enables beaming of fluorescence from many quantum emitters by having separated areas in the structure perform the functions of a cavity (the aperture) and the beaming (the patterned surface). Confocal scanning images of the collimated fluorescent emission We first show our experimental results on the slit–groove structures depicted in Figure 1a . The fabrication procedure for the nanometallic antennas, the method of introducing and optically exciting a plurality of QDs inside the slit and the optical analysis are described in the Methods section. 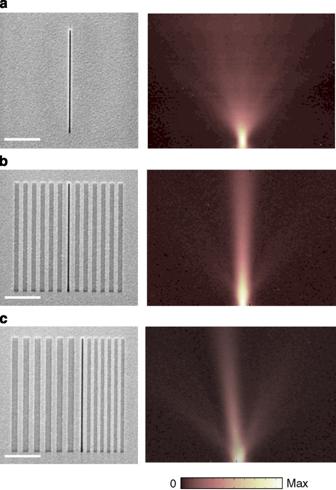Figure 2: Scanning electron microscope (SEM) images of plasmonic antennas and XZ confocal scanning images. SEM images of several plasmonic antennas and corresponding XZ confocal scanning images of the quantum dot emission. (a) A slit without side grooves. (b) A slit with side grooves optimized to produce a collimated beam normal to the metal surface (G1=G2=350 nm,g1=g2=310 nm). (c) An asymmetric slit–groove structure optimized to produce an angled beam (G1=g1=380 nm,G2=g2=320 nm). In all cases we tookW=80 nm,H=210 nm andd=30 nm. Scanning area is 20 μm in thex-direction and 15 μm in thez-direction. The white scale bar in the SEM image is 2 μm. Figure 2 shows both the scanning electron microscope images of the metallic structures and scanning confocal microscopy images of the QD emission. By performing a confocal microscopy scan in the XZ plane passing through the centre of the slit, one can visualize the beaming in blur-free images of the QD emission above the metal surface (Methods and Supplementary Methods ). We compared three cases: a slit without side grooves (a), a slit with symmetrically placed side grooves that were optimized for beaming (b) and a slit with asymmetrically placed side grooves (c). The geometrical parameters of the side grooves were optimized through numerical simulations to produce a desired flow of the light ( Supplementary methods ). Figure 2a shows that the emission from QDs in a slit without side grooves is diffracted into a broad range of angles, as expected for the emission from a subwavelength aperture. However, Figure 2b shows that a collimated beam can be produced by choosing optimized groove parameters. This geometrical optimization ensures that the planar SPPs decouple with the right phases to produce a narrow central beam by means of constructive interference. Furthermore, the structure effectively suppresses the formation of emission side lobes. Figure 2c shows the off-axis collimation of the QD emission using asymmetric slit–grooves. We achieved unprecedentedly small divergence angles of 11.5° and 11.3° for the symmetric and asymmetric slit–groove structures, respectively. Vertical collimation of the QD emission was also verified by direct Fourier-plane imaging, and this technique is compared with the confocal real-space imaging technique in the Supplementary information . For all of the antenna structures, a substantial decrease in the QD emission lifetime was observed as compared with QDs placed on a quartz substrate (Purcell effect), and it was found that the change in lifetime was strongly correlated to the central slit width ( Supplementary Methods ). Figure 2: Scanning electron microscope (SEM) images of plasmonic antennas and XZ confocal scanning images. SEM images of several plasmonic antennas and corresponding XZ confocal scanning images of the quantum dot emission. ( a ) A slit without side grooves. ( b ) A slit with side grooves optimized to produce a collimated beam normal to the metal surface ( G 1 = G 2 =350 nm, g 1 = g 2 =310 nm). ( c ) An asymmetric slit–groove structure optimized to produce an angled beam ( G 1 = g 1 =380 nm, G 2 = g 2 =320 nm). In all cases we took W =80 nm, H =210 nm and d =30 nm. Scanning area is 20 μm in the x -direction and 15 μm in the z -direction. The white scale bar in the SEM image is 2 μm. Full size image Analysis of the plasmonic beaming The observed beaming agrees quantitatively with our numerical near-to-far-field calculations ( Supplementary Fig. S5 ). The calculated wavelength dependence of the beam divergence and antenna directivity shows that narrow angle collimation can be attained over a reasonable bandwidth, covering most of the QD emission. We also found that the slit-to-first-groove distance ( g ) has a critical role in controlling the directivity of the beamed emission. Supplementary Figure S5c shows that the calculated directivity of the centre lobe (for example, directivity at θ =0°) oscillates as the magnitude of g is increased. One period of this oscillation is comparable to the SPP wavelength ( ∼ 380 nm) on the metal surface, which again confirms that the SPP propagation on the top metal surface has a key role in the beam formation [26] . The magnitude of g determines the phase that SPPs pick up in travelling from the central slit to the first groove. When g is augmented by integer numbers of SPP wavelengths, we obtain the same phase shift (modulo 2 π ) and the vertical collimation reappears. 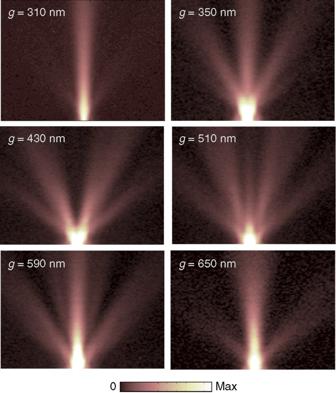Figure 3: Confocal scanning images of the QD emission for different slit-to-first-groove distances. For the images, the distancegranging from 310 to 650 nm. Strong vertical collimation of QD emission is seen forgvalues of 310 and 650 nm.G1=G2=350 nm. Figure 3 experimentally shows that a gradual increase in g from 310 to 650 nm produces various kinds of QD emission diffraction patterns. The patterns result from the complex interference of the light emerging from the slit and grooves. In agreement with our numerical results, high directivity beaming is experimentally observed at both 310 and 650 nm. Figure 3: Confocal scanning images of the QD emission for different slit-to-first-groove distances. For the images, the distance g ranging from 310 to 650 nm. Strong vertical collimation of QD emission is seen for g values of 310 and 650 nm. G 1 = G 2 =350 nm. Full size image Two-dimensional collimation of QD emission The slit–groove structure only collimates QD emission in one direction (that is, the x -direction) and a number of applications may require collimation in two directions. To achieve complete (that is, two-dimensional) collimation of QD emission, we extended our experiment to the hole–groove structures. 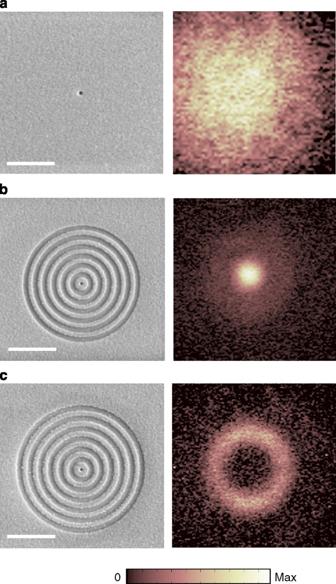Figure 4: Scanning electron microscope (SEM) images of circular plasmonic antennas and scanning confocal photoluminescence images. SEM images of several circular plasmonic antennas and corresponding scanning confocal photoluminescence images of the quantum dot photoluminescence taken in a plane 10 μm above the patterned metal surface. SEM images andXYconfocal scanning of the QD emission atZ=10 μm for (a) single hole without side grooves; (b) antenna with a concentric groove structure optimized for generating a collimated beam (G=350 nm); and (c) hole–groove structure with a larger groove spacing (G=420 nm). The central hole diameter is∼120 nm. The white scale bar in the SEM image is 2 μm. The confocal scanning size is 15 μm in both theXandYdirections. Figure 4 shows scanning electron microscope images of such structures and corresponding scans of the QD emission measured in an XY -plane 10 μm above the metal surface. As expected, the QD emission from the small (120 nm diameter) hole again diverges into a wide range of angles, producing a large beam diameter 10 μm above the patterned metal ( Fig. 4a ). However, when the same hole is surrounded by optimized side grooves ( G =350 nm), we can collimate the QD emission into a pencil-like beam, generating a small spot in the confocal image ( Fig. 4b ). It is interesting to note that the groove spacing is practically the same as for the linear grating structures that produce collimated beams. The measurements produce divergence angles of 11.7° and 11.6° in the X and Y directions. For side grooves with a larger spacing (for example, G =420 nm), we even observe a ring pattern in the QD emission ( Fig. 4c ). This is consistent with the observations made for the linear slit–groove structures with the same groove spacing ( G 1 = G 2 =420 nm; there we observed two clear side emission lobes making a 'V' shape in the XZ plane, see Supplementary Fig. S11 ). This turns into a cone of emission (by rotating the 'V') for the azimuthally symmetric hole–groove structure. Figure 4: Scanning electron microscope (SEM) images of circular plasmonic antennas and scanning confocal photoluminescence images. SEM images of several circular plasmonic antennas and corresponding scanning confocal photoluminescence images of the quantum dot photoluminescence taken in a plane 10 μm above the patterned metal surface. SEM images and XY confocal scanning of the QD emission at Z =10 μm for ( a ) single hole without side grooves; ( b ) antenna with a concentric groove structure optimized for generating a collimated beam ( G =350 nm); and ( c ) hole–groove structure with a larger groove spacing ( G =420 nm). The central hole diameter is ∼ 120 nm. The white scale bar in the SEM image is 2 μm. The confocal scanning size is 15 μm in both the X and Y directions. Full size image Active control over fluorescent emission The proposed structures for the first time enable optical antennas to serve simultaneous electronic and optical functions [27] . The patterned metal pads that produce a well-defined optical beam can at the same time be used as electrical contacts. Using such contacts, one can electrically pump a light-emitting device [28] , [29] , [30] , apply electric fields across electro-optic materials to modulate an optical signal [31] or even initiate electro-chemical reactions. Here, we demonstrate how electric fields can be applied across the central slit of our beaming structures to tune the emission wavelength and intensity of QDs by means of the quantum-confined Stark effect [32] , [33] and luminescence quenching ( Supplementary Methods ). 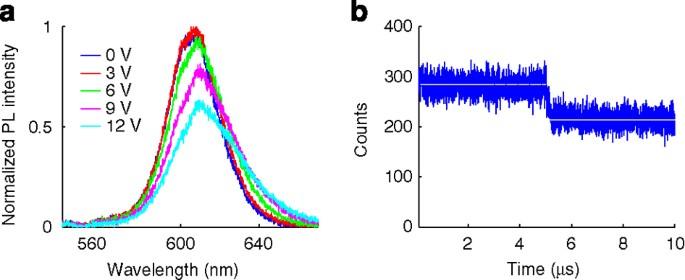Figure 5: Active control over QD emission. (a) When a DC bias voltage is applied across the gap (W=60 nm), the QD emission spectrum is seen to red shift and the overall photoluminescence signal was reduced. (b) The time-resolved histogram of QD emission intensity. The modulated square-wave signal (0–10 V, 100 kHz, 50% duty cycle) is applied. QD emission intensity is dynamically modulated with an external voltage signal. Figure 5a shows the voltage-dependent QD emission spectrum measured from our slit–groove sample. When a field is applied across the gap, the QD emission spectrum exhibits a noticeable red shift and a decrease in intensity. The spectral red shift initially increases quadratically with voltage and saturates at larger voltages ( Supplementary Fig. S9 ) as expected for the Stark effect. The intensity drop is partly attributed to field-induced dissociation of electron–hole pairs and their subsequent participation in non-radiative recombination processes [34] , [35] (such as Auger recombination). From our numerical simulations, we find that the central beam for the asymmetric slit-groove structure ( Fig. 2c ) is shifted only by 0.5° with a wavelength shift of 5 nm, which can reasonably be obtained by the Stark effect in our QDs. These shifts are too small to contribute noticeably to the observed intensity changes, but perhaps using other materials exhibiting larger wavelength tunability active beam-steering devices may be realized in the future. Figure 5: Active control over QD emission. ( a ) When a DC bias voltage is applied across the gap ( W =60 nm), the QD emission spectrum is seen to red shift and the overall photoluminescence signal was reduced. ( b ) The time-resolved histogram of QD emission intensity. The modulated square-wave signal (0–10 V, 100 kHz, 50% duty cycle) is applied. QD emission intensity is dynamically modulated with an external voltage signal. Full size image It was verified that the spectral shifts are rapidly reversible by using an alternating external voltage at 100 kHz. Figure 5b shows the time-resolved trace of the modulated QD emission near 600 nm. A modulated square-wave signal was applied across the gap with a function generator, and the QD emission was detected in a time-resolved measurement ( Supplementary Fig. S10 ). The observation of a clear modulation step verifies the ability to dynamically modulate the QD emission with an external voltage. It is expected that significantly higher modulation speeds can be realized through a careful device/system design. This opens up new opportunities for electrically modulated optical antenna devices for lighting and nanoscale spectroscopy applications. The presented results demonstrate that new optical and electrical functionalities can be obtained by simply patterning a metallic film. Patterned metal surfaces enable many simultaneous functions in the same structure, including polarization control [18] , electrical control over the emission spectrum, quantum efficiency and decay rate enhancements through the Purcell effect, optical beam-splitting ( Supplementary Fig. S11d ) and an unprecedented control over the beam directivity. We expect that similar vertical beaming can be achieved for other optical processes involving dipolar emission (such as non-linear harmonic generation, Raman scattering used frequently in spectroscopy and so on). Whereas experimentally we have only investigated emission from QD ensembles, our results implicate that optical beaming also works for a single emitter. The experimentally observed collimated beams from QD ensembles can only be formed if the emission from each individual QD is beamed in exactly the same way. The use of small metal apertures is also ideal for isolation and excitation of single emitters. The ability to direct and manipulate light emission in this manner can greatly improve the collection efficiencies. On the basis of the versatility of the described antenna structure and its unprecedented ability to produce high-directivity, electrically controllable, optical beams in one or more desired directions, we anticipate a myriad of practical and fundamental applications in optical spectroscopy, sensing, quantum optics (for example, novel single photon sources), analytical chemistry, medicine, non-linear optics, solid-state light emitters, perhaps even nanolasers [36] , [37] , [38] , [39] , and optoelectronics. After the submission of our manuscript, another group also demonstrated beaming with a circular grating and the results are consistent with our results shown in Figure 4 (ref. 40 ). Sample fabrication The optical antenna structures described in this paper were patterned into a 210-nm-thick metal film deposited onto a smooth quartz substrate. This thickness produces a resonant condition for the gap SPPs propagating up and down in the slit (z-direction). The central slits/holes and side grooves were carved into the metal by focused ion beam milling. The central slits or holes were milled entirely through the metal film. The depth of the side grooves was carefully controlled by employing a silver (30 nm)/aluminium (40 nm)/silver (140 nm) multilayer. Because aluminium exhibits a focused ion beam milling rate that is roughly five times slower than that for silver, we could use the aluminium layer as a milling stop to reproducibly obtain the target depth of the grooves ( d =30 nm). The side grooves formed gratings with a 50% duty cycle. The detailed choices for the groove dimensions and spacings followed from numerical simulations. A very thin layer ( ∼ 15 nm) of colloidal CdSe/ZnS core/shell QDs mixed with polymethylmethacrylate was spin-coated on top of the patterned metals. The scanning electron microscope image of the infiltration of the polymethylmethacrylate into the slit and side grooves is shown in Supplementary Figure S2b . Afterwards, a much thicker ( ∼ 340 nm) polymer layer (poly-vinyl alcohol) was applied by spin-coating. This layer does not mix with the bottom polymethylmethacrylate layer and provides a smooth, index-matched top-dielectric layer. Experimental setup An optical pump beam from an Ar + ion laser operating at 514 nm was directed through the quartz slide. The laser beam was purposely polarized parallel to the slit so that laser light was dramatically attenuated in the slit and the QDs inside the slit were dominantly excited over those on the top metal surface [18] . The ability to selectively confine the excitation of quantum emitters to a nanoscale volume is a real advantage and can, for example, be utilized in monitoring diffusion of single molecules into the nanoscale slit or hole, as elegantly shown by Levene et al . [41] That the photoluminescence signal was originating from the QDs inside the slit was confirmed by showing a strong dependence of several parameters on slit width, including a photoluminescence lifetime decrease through the Purcell effect, a polarization of the emission normal to the slit due to the preferential coupling of the emitters to a single-gap SPP mode, and the ability to shift the emission spectrum through the quantum-confined Stark effect. Scanning confocal microscopy is ideally suited to image optical beams [42] , [43] and we used this technique now to 'visualize', for the first time, the beaming of QD emission. Confocal images were made by scanning an ×100, 0.9 numerical aperture (NA) microscope objective above the metal surface and by collecting the QD emission through a confocal pinhole ( Supplementary Fig. S3 ). Confocal microscopy collects light from a diffraction-limited focal spot (that is, 'point' detection). By scanning a microscope objective above the sample, we can raster scan this focal spot continuously through the emitted beam and map out the radiation pattern. The obtained confocal real-space images are also compared with those from direct Fourier plane imaging ( Supplementary Fig. S6 ). Each point in a QD emission image was acquired by integrating the signals from the QD emission band. To ensure that the collected light is from the QDs only, we filtered out the illuminating laser beam at 514 nm with a notch filter and used a monochromator to spectrally select the emission from the QDs in the range 590–650 nm only. The voltage-dependent QD emission measurement ( Fig. 5 ) was performed at liquid nitrogen temperature, while all the other measurements were executed at room temperature. More information on specific calculations and measurements is provided in the Supplementary information . How to cite this article: Jun, Y. C. et al . Plasmonic beaming and active control over fluorescent emission. Nat. Commun. 2:283 doi: 10.1038/ncomms1286 (2011).